Surfactant-assisted chemical vapour deposition of high-performance small-diameter GaSb nanowires Although various device structures based on GaSb nanowires have been realized, further performance enhancement suffers from uncontrolled radial growth during the nanowire synthesis, resulting in non-uniform and tapered nanowires with diameters larger than few tens of nanometres. Here we report the use of sulfur surfactant in chemical vapour deposition to achieve very thin and uniform GaSb nanowires with diameters down to 20 nm. In contrast to surfactant effects typically employed in the liquid phase and thin-film technologies, the sulfur atoms contribute to form stable S-Sb bonds on the as-grown nanowire surface, effectively stabilizing sidewalls and minimizing unintentional radial nanowire growth. When configured into transistors, these devices exhibit impressive electrical properties with the peak hole mobility of ~200 cm 2 V −1 s −1 , better than any mobility value reported for a GaSb nanowire device to date. These factors indicate the effectiveness of this surfactant-assisted growth for high-performance small-diameter GaSb nanowires. In the past decade, due to intriguing physical properties, one-dimensional (1D) semiconductor nanowires (NWs) have attracted attention as fundamental building blocks for next-generation electronics, optoelectronics, photovoltaics and so on [1] , [2] , [3] , [4] , [5] , [6] , [7] , [8] . Although significant progress has been made in the manipulation of NW nucleation and composition in both binary and ternary systems [9] , [10] , it is still challenging to control the morphology and size of NWs on length scales ranging from the atomic upwards, particularly for the technologically important III-Sb NWs. In general, the growth of III-Sb NWs has proven difficult from small-diameter catalyst particles in various chemical vapour deposition (CVD) techniques [11] , [12] , [13] and others, yielding larger diameters than the corresponding III-As NWs [14] , [15] , [16] . This is mainly because of the required high precursor partial pressures and large atomic size of Sb. Specifically, during the CVD process, the Sb supersaturation in the catalyst particle is significantly reduced in the small diameter particles as a result of the Gibbs–Thomson effect; therefore, thin NWs can be only grown from particles with substantially higher precursor concentrations [14] . At the same time, the large atomic size of Sb would induce the surfactant effect, where Sb tends to float on top of the growing surface [17] , strongly influencing the surface or interfacial energy and reducing the migration length of adatoms. As a result, all of these factors inevitably yield the uncontrolled radial (that is, vapour–solid, VS) growth of III-Sb NWs and limit the minimum attainable diameter. To date, few studies have focussed on the synthesis of very thin (below a few tens of nanometres) III-Sb NWs owing to the difficulties caused by the above-mentioned low-vapour pressure and surfactant effects; however, the thin NW geometry is essential for many improved device applications. For example, miniaturized InSb NWs have just been demonstrated for the generation and detection of Majorana fermions [18] , [19] , [20] . GaSb NWs are of great interest for single hole transistors in spintronics and high-performance device structures in electronics [15] , [16] , [21] , where the small diameter could reduce the carrier thermalization and enhance the performance by better gate electrostatic coupling as well as less scattering. In this regard, minimizing the uncontrolled radial NW growth via the manipulation of corresponding surface energies is an important step towards the practical implementation of III-Sb NW devices with the optimized performance. Recently, it was found that, by employing the higher Sb partial pressures and heterostructure system, the Sb supersaturation in the catalyst particle could be governed such that the NW diameter was successfully reduced down to 32 nm for GaSb grown on 21 nm InAs stems [14] . A further increase in the Sb pressure was found to result in increased radial growth without reducing the NW diameter. In the present study, we explore the use of surfactant (sulfur) for the CVD growth of NWs in order to achieve very thin GaSb NWs with the diameter down to 20 nm. In contrast to the surfactant effect typically reported in the liquid phase [22] , [23] , [24] , [25] , [26] , [27] (for example, solvothermal and hydrothermal) and thin-film technologies [28] , the sulfur atoms, commonly used for the surface passivation of III–V semiconductors [29] , [30] , [31] , [32] , are contributed to form S-Sb bonds on the as-grown NW surface, effectively stabilizing the sidewalls and thus minimizing the unintentional radial growth. Importantly, the obtained NWs are highly stoichiometric, single-crystalline with a smooth surface and very uniform in diameter without any tapering. When configured into NW back-gate field-effect transistors (FETs), these devices exhibit the impressive electrical properties with I ON / I OFF ratio >10 4 , ON current density of ~50 μA μm −1 and peak field-effect mobility of ~200 cm 2 V −1 s −1 , the best mobility value reported for any GaSb NW devices to date. This superior device performance together with the low-cost surfactant-assisted NW growth on amorphous substrates holds the promise of very thin III-Sb NWs for a wide range of future technological applications. Surfactant-assisted CVD The conventional GaSb NW growth without utilizing the sulfur surfactant is optimized and directly grown by solid-source CVD on amorphous Si/SiO 2 substrates as reported before [12] , that is, 1.0 g GaSb powder as source material, 1.0-nm-thick Au film as catalyst, source temperature of 850 °C, substrate temperature of 620 °C, H 2 gas flow rate at 50 sccm and growth duration for 0.5 h. Here non-epitaxial NW growth is employed to obtain high growth yield for the subsequent potential device integration as well as to eliminate the need of underlying expensive crystalline substrates. As shown in Fig. 1a , the obtained NWs are very long (>10 μm), straight, dense and relatively thick in diameter (219±53 nm). On the contrary, adopting the sulfur surfactant, the obtained NWs become much thinner (28±9 nm) with the exact same starting catalyst thickness and growth condition ( Supplementary Fig. 1 ). In order to further reduce the NW diameter, the sulfur-assisted growth is additionally optimized using 0.5 g GaSb and 0.5 g sulfur powders as source material, 0.1-nm-thick Au film as catalyst, source temperature of 750 °C, substrate temperature of 550 °C and gas flow rate at 200 sccm. This way, the resulted NWs are even thinner with a narrower diameter distribution of 24±4 nm ( Fig. 1b ), where it is quantitatively obtained by the statistic of >100 NWs in the transmission electron microscope (TEM) images ( Fig. 1c ). This relatively small diameter and narrow distribution clearly show the advantage of this surfactant-assisted GaSb NW growth. It should also be noted that more than 90% of NWs are grown in the diameter range of 20–30 nm using sulfur as the surfactant, which would later yield a smaller variation in their corresponding electrical properties, facilitating further electronic device applications. At the same time, all as-prepared NWs are existed in the zinc-blende crystal structure of GaSb, having a = b = c =0.6095, nm (JCPDS Card No. 07-0215), based on the typical XRD patterns as depicted in Supplementary Fig. 1 . The phase purity of obtained GaSb NWs is high as there is no indication of the presence of other phases such as those of the hexagonal wurtzite phase of GaSb or phases of Sb x O y and Ga x O y . 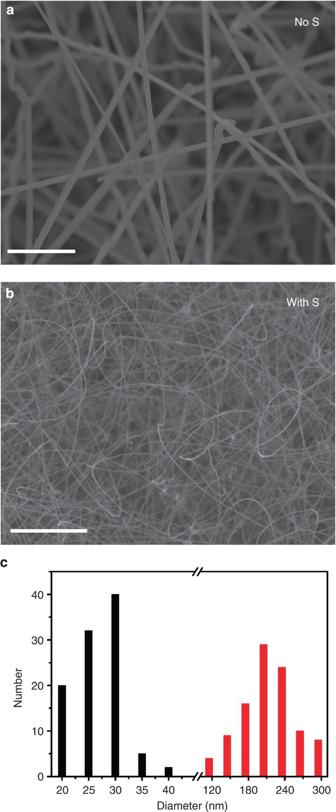Figure 1: Diameter comparison of GaSb NWs grown with and without the sulfur surfactant. (a) SEM image of the NWs grown without the surfactant. (b) SEM image of the NWs grown with the surfactant. (c) Diameter distribution of NWs grown with (black histogram, 24±4 nm) and without (red histogram, 219±53 nm) the surfactant. All the scale bars are 2 μm. Figure 1: Diameter comparison of GaSb NWs grown with and without the sulfur surfactant. ( a ) SEM image of the NWs grown without the surfactant. ( b ) SEM image of the NWs grown with the surfactant. ( c ) Diameter distribution of NWs grown with (black histogram, 24±4 nm) and without (red histogram, 219±53 nm) the surfactant. All the scale bars are 2 μm. Full size image To further assess the crystallinity and chemical stoichiometry of the as-grown sulfur-assisted GaSb NWs, high-resolution TEM and energy-dispersive X-ray spectroscopy (EDS) are performed as illustrated in Fig. 2 . Specifically, the high-resolution transmission electron microscope image of the NW catalyst/body region ( Fig. 2a ) explicitly shows the lattice of the spherical catalytic seed as well as the body, inferring a vapour–liquid–solid (VLS) or vapour–solid–solid growth mode. In addition, there is an amorphous layer of ~2 nm around the NW body, which is always observed in the literature [33] , [34] . On the basis of the high-resolution transmission electron microscope imaging and corresponding reciprocal lattice spots extracted by fast Fourier transform, the NW has a catalyst/NW interface orientation relationship of cubic AuGa 2 {111}|cubic GaSb{111}, without any noticeable amount of crystal defects such as stacking faults or inversion domains, and so on. The grown NWs have the dominant growth axis of <111> as this growth direction involves the lowest free energy crystal planes and thus are more thermodynamically favourable [35] , [36] , while a small amount of NWs with <110> direction are also observed, which is probably induced by the defect formation in the initial stage of the NW growth, favouring the next higher index directions [17] . The AuGa 2 catalyst is then verified by the EDS results ( Fig. 2b ) of the catalyst tip in the point P1 with an Au:Ga ratio of ~1:2, and the NW body has a balanced stoichiometry of Ga:Sb~1:1 in point P2. Although there is not any significant amount of sulfur signal in the P2 spectra, it does appear in the elemental mapping with sufficiently long acquisition time ( Fig. 2c–f ), in which the uniform distribution of Ga, Sb, Au and S atoms along the NW body is illustrated. All of these demonstrate the well-controlled surface morphology, crystallinity and balanced stoichiometry of GaSb NWs (within the resolution of EDS (~1%), excluding the existence of any Ga or Sb clusters) achieved with this sulfur-assisted CVD technique. 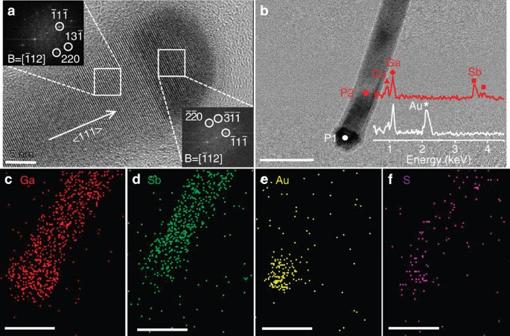Figure 2: Electron microscopy characterization of surfactant-assisted grown GaSb NWs. (a) High-resolution transmission electron microscope (HRTEM) image and corresponding fast Fourier transform (FFT) of a representative NW, illustrating the catalyst seed/body region. The diameter is ~23 nm with the growth direction of <111>. Scale bar is 5 nm. (b) TEM image and the corresponding EDS spectra obtained on the catalyst tip (P1) and the NW body (P2). Scale bar is 50 nm. (c–f) EDS elemental mappings of Ga, Sb, Au and S, respectively. Scale bars are 30 nm. Figure 2: Electron microscopy characterization of surfactant-assisted grown GaSb NWs. ( a ) High-resolution transmission electron microscope (HRTEM) image and corresponding fast Fourier transform (FFT) of a representative NW, illustrating the catalyst seed/body region. The diameter is ~23 nm with the growth direction of <111>. Scale bar is 5 nm. ( b ) TEM image and the corresponding EDS spectra obtained on the catalyst tip (P1) and the NW body (P2). Scale bar is 50 nm. ( c – f ) EDS elemental mappings of Ga, Sb, Au and S, respectively. Scale bars are 30 nm. Full size image Roles of the surfactant and its effect on NW growth It should be noted that the EDS signal of sulfur only indicate the existence of sulfur atoms in the NWs, but not the exact location of them such as either incorporating on the NW surface or doping within the NW core. In order to determine the accurate position of these sulfur atoms, thickness-dependent X-ray photoelectron spectroscopy (XPS) studies are performed to assess the elemental composition and chemical state of all constituents along the NW radial direction. Here the surface layers of NWs can be removed by first treating them in the mild oxygen plasma (50 W, 30 s) and then etching them in the dilute HF solution (1%, 30 s) followed by the thorough DI water rinse. As presented in Fig. 3 , after the etching, there are still dense NWs with smooth surface on the substrates. Notably, the average diameter of processed NWs is reduced from the original value of ~24 to ~18 nm, which indicates the outmost surface layer (~3 nm in thickness) of the as-prepared NWs can be completely removed by this treatment of oxygen plasma and HF etching. Although the treatment of oxygen plasma and HF etching can also yield smaller diameter NWs, their corresponding NW electrical performance would be degraded substantially because of the increased surface states resulted in this etching (see details in Supplementary Fig. 2 ), indicating this post-growth etching process as an inappropriate method for the fabrication of small diameter NWs as compared with our surfactant-assisted growth technique. 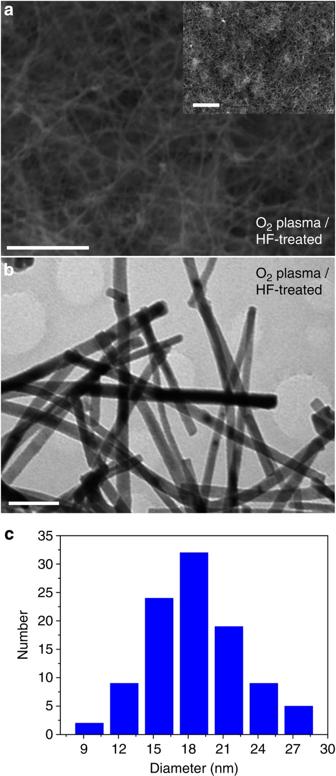Figure 3: Diameter statistics of GaSb NWs processed with oxygen plasma treatment and dilute HF etching. (a) SEM image of the processed NWs (scale bar of the inset is 2 μm). Scale bar is 500 nm. (b) TEM images of the processed NWs. Scale bar is 100 nm. (c) Diameter distribution (blue histogram, 18±4 nm) obtained from >100 NWs characterized in the corresponding TEM images. Scale bar is 50 nm. Figure 3: Diameter statistics of GaSb NWs processed with oxygen plasma treatment and dilute HF etching. ( a ) SEM image of the processed NWs (scale bar of the inset is 2 μm). Scale bar is 500 nm. ( b ) TEM images of the processed NWs. Scale bar is 100 nm. ( c ) Diameter distribution (blue histogram, 18±4 nm) obtained from >100 NWs characterized in the corresponding TEM images. Scale bar is 50 nm. Full size image As shown in Fig. 4 , XPS spectra of the NWs before (that is, with S, black curve) and after the oxygen plasma/HF treatment (that is, treated, blue curve) are all calibrated with the C1 s peak. The relatively small shifting of the spectra might be attributed to size effect as reported in the literatures [37] , [38] , [39] , which is not emphasized herein. The NWs grown without the sulfur surfactant are also measured as the control sample (that is, no S, red curve). In any case, the S 2 s (binding energy ~226.6 eV) spectra given in Fig. 4a clearly indicate that S is only observed in the sample before the treatment but not in the ones after the treatment and the control sample. This designates that the S atoms only exist and incorporate in the surface layer of the as-prepared NWs grown with the sulfur surfactant, in which these S-containing surface layer is effectively removed by the oxygen plasma/HF treatment. The XPS spectra of Ga 3 d ( Fig. 4b,c ) and Sb 4 d ( Fig. 4d-f ) are also collected to explore the chemical bonding state of the surface sulfur atoms. In the Ga 3 d spectra depicted in Fig. 4b , two peaks centred at 19.23 and 20.93 eV are observed for the NWs grown with (black curve) and without (red curve) the sulfur surfactant, attributing to the GaSb and Ga-O bonds, respectively. Similar results are obtained by Gauss–Lorentz decomposing the Ga 3 d spectrum of the process treated NWs as shown in Fig. 4c (blue curve), inferring that S atoms are not bonded to Ga. On the other hand, based on the peak fit of Sb 4 d spectra ( Fig. 4e ) of the NWs with S (black curve), chemical bonds of Sb-Ga (3/2 at 31.78 eV, 5/2 at 33.01 eV), Sb-S (34.22 eV) and Sb-O (35.37 eV) are all observed, while only Sb-Ga and Sb-O bonds are found in the NWs grown without S (red curve) and process treated (blue). As a result, one can deduce obviously that the S atoms are connected with Sb atoms to form covalent bonds of Sb-S on the NW surface. This way, it can be understood that S performs as an effective surfactant with the function of stabilizing the surface Sb atoms, inhibiting the uncontrolled NW radial growth to give very thin and uniform GaSb NWs here. 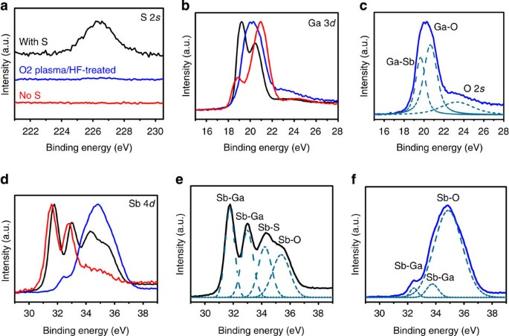Figure 4: Surface elemental analysis of GaSb NWs. (a) S 2sbonding region. (b,c) Ga 3dbonding region. (d–f) Sb 4dregion. (c,e,f) Gauss–Lorentz fitted spectra of the Ga 3dbonding region of the treated NWs, Sb 4dbonding region of the S-assisted NWs before and after the treatment with a correlation coefficient ofr2>0.99, respectively. (Black, blue and red curves are the X-ray photoelectron spectroscopy (XPS) spectra of GaSb NWs prepared with S, GaSb NWs grown with the sulfur surfactant and processed with oxygen plasma treatment as well as dilute HF etching, and the control sample of GaSb NWs grown without the sulfur surfactant, respectively). Figure 4: Surface elemental analysis of GaSb NWs. ( a ) S 2 s bonding region. ( b , c ) Ga 3 d bonding region. ( d – f ) Sb 4 d region. ( c , e , f ) Gauss–Lorentz fitted spectra of the Ga 3 d bonding region of the treated NWs, Sb 4 d bonding region of the S-assisted NWs before and after the treatment with a correlation coefficient of r 2 >0.99, respectively. (Black, blue and red curves are the X-ray photoelectron spectroscopy (XPS) spectra of GaSb NWs prepared with S, GaSb NWs grown with the sulfur surfactant and processed with oxygen plasma treatment as well as dilute HF etching, and the control sample of GaSb NWs grown without the sulfur surfactant, respectively). Full size image Moreover, as depicted in Fig. 4b , the relative intensity of the Ga-O peak of the NWs without S (red curve) is significantly higher than that of the NWs with S (black curve). In addition, there is a much smaller tail peak related to Sb-O in the Sb 4 d spectra ( Fig. 4d ) of the NWs without S (red curve) as compared with the one with S (black curve). All these suggest that the NWs grown without the sulfur surfactant consist of a Ga x O y -rich surface layer, while the NWs grown with S come with the more uniform Ga x O y and Sb x O y oxide layers. This is in accordance with the growth kinetics in this solid-source CVD that the Sb supply would be deficient from the solid source in the final growth step because of its relatively higher vapour pressure as compared with that of the group III constituent, leading to the Ga-rich radial growth on the NW surface and the Ga x O y -rich surface layer in the conventional growth without the sulfur surfactant. When the sulfur is employed, it stabilizes the GaSb radial NW surface such that a more uniformly distributed oxide (Ga x O y and Sb x O y ) and Sb-S layer is obtained. At the same time, the sulfur atoms are found to only bond on the NW surface during the growth, instead of incorporating into the NW core for doping. This is probably owing to the low solubility of sulfur in the Au-Ga catalyst seeds as well as its relatively high vapour pressure. This way, these S atoms cannot be introduced easily into the grown NW core via the VLS mechanism through the catalytic tip and the tip/body interface [40] ; they prefer to accumulate on the NW surface and passivate the active Sb sites, being consistent to the observed XPS results. The surfactant effect of sulfur in inhibiting the radial growth of GaSb NWs by passivating the surface Sb site is further ascertained by the comparison of TEM images in Fig. 5 . 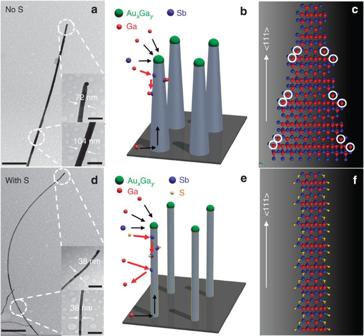Figure 5: Growth mechanisms of GaSb NWs obtained with and without the use of sulfur surfactant. (a,d) TEM images of representative NWs grown without and with the use of surfactant, respectively (scale bars are all 200 nm in the insets). Scale bars are 1 μm. (b,c) Schematic illustration and corresponding atomic model depiction of the conventional VLS NW growth mode, accordingly. (e,f) Schematic demonstration and corresponding atomic model illustration of the surfactant-assisted VLS NW growth scheme, respectively. Figure 5a shows an obvious tapering of ~5 nm μm −1 along the length of a representative NW grown without the use of sulfur, while the diameter is extremely uniform along the entire length (>10 μm) of another NW grown with the surfactant illustrated in Fig. 5d . In order to demonstrate the effect of sulfur in this CVD process in details, growth schematics and corresponding atomic models are also given and contrasted ( Fig. 5 ). It is well known that the catalytic particle size plays an important role in controlling the NW diameter. In order to study the effect of S on Au catalysts, the catalyst film (1 nm) is annealed with S at 550 °C for 10 min. As a comparison, the annealing process is also performed without S. After annealing, the size distribution of Au particles is then assessed using AFM. As presented in the Supplementary Fig. 3 , it is obvious that a similar average particle diameter is obtained, indicating that sulfur plays an insignificant role on the formation of Au catalytic particles. One should also notice that NWs can grow very thick using these small Au nanoparticles as the catalyst without S surfactant, inferring that the Au nanoparticles may aggregate to form larger particles during the NW nucleation, which might not happen in the process using S surfactant. However, controlling this particle aggregation is not the key in this thin NW growth, as evidenced in our control experiments. Specifically, we first anneal the Au catalyst with S, stop the growth to remove S and then continue the NW growth without any S, which results in no NW growth (it showed a similar morphology with the samples prepared without any sulfur, see Supplementary Fig. 4a ). Figure 5: Growth mechanisms of GaSb NWs obtained with and without the use of sulfur surfactant. ( a , d ) TEM images of representative NWs grown without and with the use of surfactant, respectively (scale bars are all 200 nm in the insets). Scale bars are 1 μm. ( b , c ) Schematic illustration and corresponding atomic model depiction of the conventional VLS NW growth mode, accordingly. ( e , f ) Schematic demonstration and corresponding atomic model illustration of the surfactant-assisted VLS NW growth scheme, respectively. Full size image After the NW nucleation, during the VLS growth, the Au catalyst is melted and becomes small liquid droplets on the substrate at high temperatures. In addition, the GaSb powder is decomposed into precursor vapours and carried towards the substrate by the H 2 flow. In an ideal case, Ga atoms would chemically react and be incorporated into the grown NWs through the Au x Ga y catalytic nanotip, while Sb atoms would react to induce NW growth at the interface between the nanotip and the body. This way, NWs with the smooth surface and uniform diameter would be prepared. Realistically, during the growth process, it is inevitable that Ga will also be surface-diffused from the NW base and reacted with the surface-terminated Sb, contributing to the unintentional radial (VS) NW growth (red arrow); as a result, the tapering and non-uniform NW diameter (white circle) are obtained ( Fig. 5b,c ), as commonly found in other III–V NW growth [9] , [40] , [41] , [42] , [43] , [44] . With the aid of sulfur surfactant passivating these surface active Sb sites, the NW sidewall is stabilized (red arrow) and minimal uncontrolled radial growth results ( Fig. 5e,f ). In this case, very thin GaSb NWs with a uniform diameter and smooth surface can then be achieved by adopting this simple sulfur surfactant-assisted CVD process. As a result, the key effect of sulfur in this thin NW growth is to passivate the NW surface to alleviate the uncontrolled radial growth, instead of controlling the particle aggregation of the Au catalyst. Notably, the amount of sulfur surfactant is also expected to play a crucial role in minimizing this unwanted NW radial growth; this effect has been assessed in Supplementary Fig. 4 . In brief, when the mass of sulfur used is less than 0.5 g, very few NWs can be grown because of the inadequate Sb supersaturation in the small-diameter catalyst particles. On the other hand, when the mass of sulfur is larger than 0.5 g, dense NWs are obtained, but with a significant amount of kinks and are not straight, owing to the overloading of excess sulfur on the NW surface. Their corresponding NW electrical performance will be discussed in detail in the subsequent sections. Electrical performance of fabricated NWFETs To shed light on the electrical properties of as-prepared GaSb NWs, global back-gate NWFETs are fabricated as typically shown in Fig. 6a , along with the scanning electron microscope (SEM) image of a representative NW grown with the use of sulfur surfactant. The diameter, d , is found to be ~32 nm and the channel length, L , is determined to be ~2 μm. The transfer characteristics of both NW devices (that is, grown with and without S) exhibit the typical p-type conduction ( Fig. 6b ), inconsistent with XPS results such that S atoms only play a role in passivating the NW sidewall, but do not dope into the lattice, even though S is a common n-type dopant in III–V semiconductors. It is also noted that the ON current density (~50 μA μm −1 ), OFF current (~50 pA) and I ON / I OFF ratio (>10 4 , obtained from the log scale of I DS − V GS curves in Supplementary Fig. 5 ) of the sulfur-assisted NW device are much more improved as compared with the ones of thick NWs grown without surfactant. In addition, the linear output characteristics are given in Supplementary Fig. 5 , confirming the ohmic-like contact as Ni has a higher work function (~5.2 eV) than the Fermi level of p-GaSb (<4.8 eV). 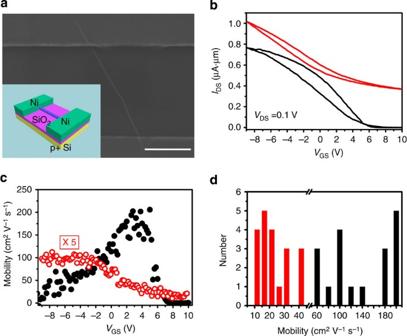Figure 6: Comparison of electrical properties of GaSb NWs obtained with and without the use of sulfur surfactant. (a) SEM image of a representative FET with the NW channel grown with the use of surfactant. Inset shows the corresponding device schematic. Scale bar is 1 μm. (b) Normalized transfer characteristics of the NW devices. (c) Mobility calculation of the corresponding NW devices. (d) Mobility distribution based on more than 40 NW devices. (Black curves are the electrical property of GaSb NWs prepared with S and red curves are the electrical property of the control sample of GaSb NWs grown without the sulfur surfactant). Figure 6: Comparison of electrical properties of GaSb NWs obtained with and without the use of sulfur surfactant. ( a ) SEM image of a representative FET with the NW channel grown with the use of surfactant. Inset shows the corresponding device schematic. Scale bar is 1 μm. ( b ) Normalized transfer characteristics of the NW devices. ( c ) Mobility calculation of the corresponding NW devices. ( d ) Mobility distribution based on more than 40 NW devices. (Black curves are the electrical property of GaSb NWs prepared with S and red curves are the electrical property of the control sample of GaSb NWs grown without the sulfur surfactant). Full size image Previously, there has been some controversy regarding the mobility calculation of nanodevices when covered by a high-κ dielectric layer and a metal top gate [45] , [46] . However, in this work, the small diameter GaSb NWFET is configured in a global back-gated geometry, and is not covered with any high-κ dielectric layer and the metal top gate. In this case, one of the well-accepted methods for the mobility determination is based on the square law model and the corresponding field-effect mobility can be calculated by using the low-bias (for example, V DS =0.1 V) transconductance in the transfer characteristics, g m =( dI DS )/( dV GS )| V DS , and the analytical expression, μ = g m ( L 2 / C OX )(1/ V DS ), where C OX is the gate capacitance obtained from the finite element analysis software COMSOL with respect to different diameters of the NW [12] , [47] . Notably, this C OX determined from the simulation gives a relatively accurate gate capacitance; together with the known NW length (in the channel of FET) and diameter, the field-effect mobility of the NW can be gained reliably [48] . The calculated peak hole mobility of a small diameter sulfur-assisted NW device is found to be ~200 cm 2 V −1 s −1 , whereas the peak hole mobility of a thick NW device (that is, no S) is only ~20 cm 2 V −1 s −1 , further proven by the statistics of 20 devices as shown in Fig. 6d . Notably, wire-to-wire variations do exist in the statistics, which may be attributable to the dependence of electrical properties on NW diameters, orientations, surface roughness and others. In any case, this significant performance enhancement is mainly because of the sulfur surfactant passivation in reducing the surface states and the better crystal quality in minimizing the crystal defects. At the same time, the hole concentration of the sulfur-assisted NW can also be estimated using the equation, n h = Q /( qπr 2 L )=( C OX V th )/( qπr 2 L ), where r is the NW radius (16 nm) and V th is the threshold voltage (~7.5 V). The concentration is estimated to be ~3.1 × 10 18 cm −3 , which is in fairly good agreement with the intrinsic undoped concentration level reported in the literature, with the free carriers originating from native crystal defects such as Ga Sb antisite or Ga vacancy. Furthermore, one should also notice that this carrier mobility is highly dependent on the carrier concentration. Although the highest hole mobility of GaSb (bulk material) is reported as ~1,000 cm 2 V −1 s −1 , it can only be reached at a hole concentration of ~10 16 cm −3 . The hole concentration of the thin GaSb NW is found to be ~3.1 × 10 18 cm −3 , which corresponds to the highest achievable hole mobility of ~400 cm 2 V −1 s −1 , not too far away from the current mobility of 200 cm 2 V −1 s −1 (ref. 49 ), probably because of the surface states that might not be fully passivated [50] . Regardless, the hole mobility of our thin GaSb NWs is the highest reported in the literature to date ( Table 1 ) and also does not vary much from their theoretical limits. Table 1 The comparison of peak mobility and other electrical properties of the p-type GaSb-nanowire field-effect transistors. Full size table It is also noticeable that there is an inverse relationship between the hole mobility and the NW diameter here, which is in distinct contrast to the typically higher mobility for thicker NWs observed in the previous NW works [48] , [51] . This unique phenomenon can be attributed to the in situ surface passivation effect of sulfur on the GaSb NW sidewall by saturating the dangling bonds of surface Sb atoms, reducing the surface state density and thus diminishing the surface scattering of holes. Alternatively, there are abundant surface states that exist on the thick NW surface grown without the surfactant, significantly scattering the hole propagation and leading to a far lower hole mobility. From the literature, sulfur is an effective passivating specie for III–V NWs, which is always introduced to the NW surface by the post-growth treatment such as the (NH 4 ) 2 S x solution dipping [32] . This in situ passivation effect of sulfur further illustrates the advantages of this surfactant-assisted CVD technique in attaining high-performance III–V NWs. In order to further ascertain the passivating effect of sulfur rather than being a dopant during the NW growth, the electrical properties of GaSb NWs prepared with additional amount of sulfur (that is, 1 g, instead of 0.5 g) are studied and illustrated in Supplementary Fig. 6 . As depicted in the SEM image ( Supplementary Fig. 4d ), dense but not straight GaSb NWs with significant amounts of kinks are obtained. When configured into NW devices ( Supplementary Fig. 6 ), it is clear that the straight NWs give a similar electrical behaviour with those grown with 0.5 g of sulfur surfactant, such as the ON/OFF current ratio and mobility; however, the electrical performance of the kinked (curved) NWs becomes poorer, yielding much lower ON current and hole mobility. It is obvious that by adding more sulfur during the growth, the obtained straight NWs still give a similar electrical performance, rather than lowering the p-channel current, indicating that the sulfur does not incorporate into the NW core as the potential n-type dopants. Adding more sulfur would only induce the kink morphology because of the sulfur agglomeration on the NW surface. Combining with our thickness-dependent XPS results, since there is no S signal detected after the outmost NW surface layer is removed, we can conclude that insignificant amounts of S are doped into the NW body. Generality of the adopted surfactant-assisted growth method Moreover, another typical III–V semiconductor (that is, GaAs) NW system is employed to demonstrate the generality of this adopted surfactant-assisted growth method. As reported in the previous work [52] , GaAs NWs with relatively short length (~3 μm) and large-diameter distribution (76.1±49.9 nm) were obtained by the solid-source CVD method utilizing 12-nm-thick Au film as the catalyst without sulfur. On the contrary, by adopting the sulfur surfactant process, the obtained GaAs NWs become much thinner with a narrower diameter distribution of 36.9±8.5 nm, as shown in Fig. 7 . At the same time, the electron energy loss spectroscopy mapping demonstrates the uniform distribution of Ga, As and S atoms along the NW body ( Supplementary Fig. 7 ). More importantly, similar to the case of sulfur surfactant growth of GaSb NWs, XPS is also performed here to confirm the elemental composition and chemical state of all constituents along the radial direction of GaAs NWs, especially the formation of covalent As-S bonds on the surface in minimizing non-uniform and tapered NWs, as well as the surface oxide formation ( Supplementary Fig. 8 ). All of these results are analogous to the case of sulfur surfactant growth of GaSb NWs, in which sulfur is employed as the surfactant with the function of stabilizing the surface group V atoms, inhibiting the uncontrolled NW radial growth to give thin and uniform NWs. Notably, these small diameter GaAs NWs also demonstrate the p-type semiconductor behaviour, consistent with previous reports [33] . In the literature, it is shown that GaAs NWs would yield different electronic behaviours with different NW diameters, in which thin GaAs NWs would give p-type conduction while thick NWs would give n-type conduction, owing to the interface trapping states existed between the intrinsic GaAs core and its amorphous oxide shell. As a result, because of the sulfur passivation on the NW surface here, the surface oxide formation and its corresponding interface trapping effect are significantly reduced and a lower ON current (less p-type) results, as compared with the GaAs NWs prepared by conventional solid-source CVD method [33] . In summary, the adopted surfactant-assisted CVD approach can also be successfully implemented for the growth of GaAs NWs, further illustrating this surfactant-assisted scheme as a versatile growth platform extending to other NW material systems. 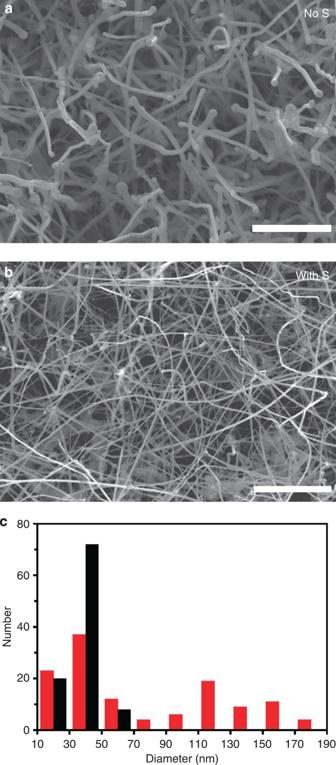Figure 7: Comparison of GaAs NWs grown with and without the sulfur surfactant. (a) SEM image of the NWs grown without the surfactant (1.0 g GaAs powder as the source material). (b) SEM image of the NWs grown with the surfactant (0.6 g GaAs powder and 0.6 g sulfur powder as the source materials). (c) Diameter distribution of NWs grown with (black histogram, 36.9±8.5 nm) and without (red histogram, 76.1±49.9 nm) the surfactant. All the scale bars are 2 μm. Figure 7: Comparison of GaAs NWs grown with and without the sulfur surfactant. ( a ) SEM image of the NWs grown without the surfactant (1.0 g GaAs powder as the source material). ( b ) SEM image of the NWs grown with the surfactant (0.6 g GaAs powder and 0.6 g sulfur powder as the source materials). ( c ) Diameter distribution of NWs grown with (black histogram, 36.9±8.5 nm) and without (red histogram, 76.1±49.9 nm) the surfactant. All the scale bars are 2 μm. Full size image Although GaSb NWs have been widely explored as promising active channel materials for various technological applications, the required performance improvement still lags behind the expectation, largely suffering from the uncontrolled radial VS growth during the NW synthesis. The current work provides experimental evidence on the effects of surfactant in the CVD growth of high-performance small-diameter GaSb NWs. Specifically, sulfur has been proven as a proper surfactant here because of its formation of stable S-Sb bonds on the NW surface, which can effectively stabilize the unsaturated surface-terminated Sb sites in order to minimize the uncontrolled radial NW growth. This way, very thin and uniform GaSb NWs with diameters down to 20 nm can be easily achieved; this contrasts with the conventional vapour–liquid–solid growth of tapered GaSb NWs. In addition, when configured into NWFETs, the electrical performance, such as the ON current density, OFF current and I ON / I OFF ratio, have been greatly improved owing to the reduced surface carrier scattering and improved crystal quality in these thin NW geometries. This surfactant-assisted CVD scheme might also be employed as a growth platform for other NW material systems, such as other typical III–V semiconductors of GaAs. In conclusion, the use of sulfur surfactant enables the growth of uniform, well-controlled, small-diameter GaSb NWs with impressive electrical properties and could open up the possibility for many practical applications. Nanowire synthesis GaSb NWs studied in this work are grown by employing the sulfur surfactant-assisted solid-source CVD with the solid GaSb (99.999% purity) and sulfur powders (99.99% purity) as the source materials. Briefly, a dual-zone horizontal tube furnace, one zone for the solid source (upstream) and one zone for the growth substrate (downstream), is used as the reactor for the synthesis of GaSb NWs (the growth set-up can be seen in Supplementary Fig. 9 ). At first, the Au thin film is pre-deposited on Si/SiO 2 substrates (50-nm-thick thermally grown) and then the substrate is placed in the middle of the downstream zone for the NW growth. The solid sources, GaSb and sulfur powders, are placed within two separate boron nitride crucibles, with distances of 15 and 9 cm away from the sample, respectively. As shown in the growth set-up, the sulfur powder is placed in the middle of the two zones. During the growth, the source and substrate are heated to the required temperatures accordingly. Hydrogen (99.9995% purity) is used as the carrier gas to transport the thermally vaporized precursors to the downstream. Before heating, the pressure of the quartz tube is pumped to 3 × 10 −3 Torr and then purged with H 2 for 0.5 h. After the growth, the source and substrate heater are stopped together and cooled to room temperature under the hydrogen flow. Material characterization Surface morphologies of the grown NWs are examined with a scanning electron microscope (Philips XL30, carried out at the City University of Hong Kong) and a TEM (Philips CM-20, carried out at the City University of Hong Kong). Crystal structures are determined by collecting XRD patterns on a Philips powder diffractometer using Cu Kα radiation ( λ =1.5406 Å) and imaging with a high-resolution TEM (JEOL 2100 F, carried out at the City University of Hong Kong). Elemental mappings are performed using an EDS detector attached to the JEOL 2100 F to measure the chemical composition of the grown NWs. The chemical state of the as-prepared GaSb NWs is examined by X-ray photoelectron spectroscopy (ULVAC-PHI5802, carried out at the City University of Hong Kong). For the TEM and elemental mappings, the NWs are first suspended in the ethanol solution by ultrasonication and drop-casted on the grid for the corresponding characterization. NWFET fabrication and measurements NWFETs are fabricated by drop-casting the NW suspension on highly doped p-type Si substrates with a 50-nm-thick thermally grown gate oxide. Photolithography is utilized to define the source and drain regions, and 50-nm-thick Ni film is thermally deposited as the contact electrodes followed by a lift-off process. The electrical performance of the fabricated back-gated FETs is then characterized with a standard electrical probe station and an Agilent 4155C semiconductor analyser (carried out at the City University of Hong Kong). How to cite this article: Yang, Z.-x. et al. Surfactant-assisted chemical vapour deposition of high-performance small-diameter GaSb nanowires. Nat. Commun. 5:5249 doi: 10.1038/ncomms6249 (2014).